Hidden one-dimensional spin modulation in a three-dimensional metal Pressure can transform a transparent material into an opaque one, quench the moments in a magnet and force solids to flow like liquids. At 15 GPa, the pressure found 500 km below the earth’s surface, the semiconductors silicon and germanium superconduct. Yet, at this same pressure, we show here that the magnetism in metallic GdSi remains completely robust even as it shrinks by one-seventh of its volume. Non-resonant X-ray magnetic diffraction in a specially designed diamond anvil cell, combined with band structure calculations, reveal the stability of the incommensurate spin density wave, which can be traced to a persistently nested portion of the Fermi surface that becomes increasingly one-dimensional under pressure. A cooperative interaction between nested, itinerant spins and local magnetic moments provides the organizing principle for the modulated magnetic order, salient both for its insights into the role of topology in ordered states and its potential functionality. One-dimensional materials display a variety of intricate collective states, from gapless Luttinger liquids with spin–charge separation to gapped, interleaved spin and charge density waves (SDWs and CDWs). Model one-dimensional organic conductors such as (TMTTF) 2 X and TTF-TCNQ [1] , [2] , [3] , [4] , [5] , [6] sit on the edge between spin and charge order and superconductivity. One-dimensional instabilities also exist within materials of higher dimension and can play a dominant role in determining their properties. For example, in the cubic A15 compound V 3 S, dense linear chains of V atoms provide an enhanced density of states at the Fermi surface, leading to an unexpectedly high superconducting transition temperature [7] . Similarly, Fermi surface nesting along particular directions in reciprocal space dominates the magnetic behaviour of three-dimensional elemental Cr [8] and the two-dimensional, rare-earth tritellurides [9] . Recently, a new mechanism for SDW order was discovered in the rare-earth intermetallic GdSi at ambient pressure. The ordering wave vector is incommensurate with both the b* - and c* -axes at Q =(0, q b , q c )~(0, 0.483, 0.092) due to a quasi-one-dimensional Fermi surface instability [10] . The antiferromagnetic state is composed of nested itinerant electrons in a cooperative interaction with localized Gd 4 f moments: the itinerant electrons satisfying the nesting condition are coupled in a SDW via scattering from the local moments, while the local moments interact through the Ruderman–Kittel–Kasuya–Yosida indirect exchange mediated by the itinerant SDW and assume the ordering wave vector determined by the nesting. This self-consistent, cooperative organization between local and itinerant spins is analogous to the interplay of lattice distortions and charge in phonon-mediated CDWs. Most SDWs and CDWs are highly susceptible to pressure [11] , [12] . However, the stability and evolution of the itinerant magnetic order as the separation between local moments is tuned in this new type of SDW has not been explored. Hydrostatic pressure P provides continuous fine-tuning capability as well as a vast range with P >300 GPa accessible in diamond anvil cells [13] . However, tracking magnetism under pressure is technically difficult and often limited to indirect or spectroscopic techniques, such as electrical transport [6] , [14] , magnetostriction, X-ray emission [15] , nuclear magnetic resonance [2] , [3] , [4] and Mossbauer. Neutron or X-ray magnetic diffraction needs to be employed for direct insight into the long-range magnetic order and the spin structure. The typical pressure range for neutron magnetic diffraction is 25 GPa for powders [16] and <10 GPa for single crystals [17] . Single-crystal X-ray magnetic diffraction has become competitive over the past decade as a direct probe of antiferromagnetism under pressure [18] , [19] , [20] . In the following sections, we present a combined experimental and theoretical approach from both non-resonant X-ray magnetic diffraction and ab initio band structure calculations to elucidate the pressure evolution of the SDW ground state in GdSi. We use newly designed, wide-angle, partially perforated diamond anvils to increase signal throughput and reduce background (Methods; Fig. 1 ). This improvement in high-pressure techniques has allowed us to track directly the SDW ground state in GdSi with quantitative measurements of both the magnetic order parameter and the wave vector for pressures up to 17 GPa. Both quantities remain stable even as the lattice varies significantly, until a first-order structural transition from monoclinic to orthorhombic occurs. Using band structure calculations, the stability of the antiferromagnetism can be traced back to a persistently nested Fermi surface, which grows more and more one-dimensional under pressure during a charge transfer process between different itinerant bands. 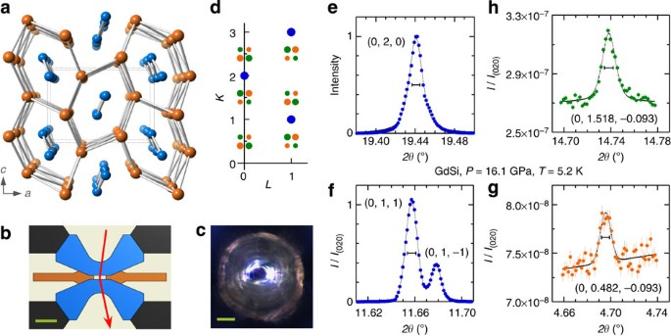Figure 1: High-pressure X-ray magnetic diffraction. (a) Lattice structure of GdSi, viewed along thebaxis, with a depth of three unit cells. All bonds between Gd (orange) and Si (blue) are removed to highlight the linear nature of double Si chains surrounded by Gd tubes. (b) A schematic of a new type of perforated diamond anvil designed for X-ray magnetic diffraction. X-rays (red lines with arrow) diffract off the sample (not shown) from inside the pressure chamber, which is constructed with two Boehler–Almax type of diamond anvils with wide-angle perforation (blue) and a gasket (orange). Scale bar, 0.8 mm. (c) Sample chamber assembly viewed through one of the perforated diamond anvils. Both sample (rectangular shadow in the middle) and silver manometer (triangular shadow) can be seen in the 400-μm diameter sample chamber. Scale bar, 0.1 mm. (d) Schematic of the diffraction patterns of both lattice (blue) and incommensurate magnetic order (orange and green) of GdSi in theK–Lplane. Orange and green colours correspond to two degenerate magnetic domains. Magnetic diffraction intensities surrounding the forbidden lattice orders such as (0, 1, 0) are much weaker. (e–h) Longitudinal scans of both lattice and magnetic order. Each peak is fit with a pseudo-Voigt function, in addition to an extra linear background for magnetic peaks (g,h). Vertical error bars represent 1σs.d. of counting statistics. The horizontal bars at the middle of each peak represent the FWHM of the instrument resolution. All intensities are normalized to that of the (0, 2, 0) Bragg peak. Figure 1: High-pressure X-ray magnetic diffraction. ( a ) Lattice structure of GdSi, viewed along the b axis, with a depth of three unit cells. All bonds between Gd (orange) and Si (blue) are removed to highlight the linear nature of double Si chains surrounded by Gd tubes. ( b ) A schematic of a new type of perforated diamond anvil designed for X-ray magnetic diffraction. X-rays (red lines with arrow) diffract off the sample (not shown) from inside the pressure chamber, which is constructed with two Boehler–Almax type of diamond anvils with wide-angle perforation (blue) and a gasket (orange). Scale bar, 0.8 mm. ( c ) Sample chamber assembly viewed through one of the perforated diamond anvils. Both sample (rectangular shadow in the middle) and silver manometer (triangular shadow) can be seen in the 400-μm diameter sample chamber. Scale bar, 0.1 mm. ( d ) Schematic of the diffraction patterns of both lattice (blue) and incommensurate magnetic order (orange and green) of GdSi in the K–L plane. Orange and green colours correspond to two degenerate magnetic domains. Magnetic diffraction intensities surrounding the forbidden lattice orders such as (0, 1, 0) are much weaker. ( e – h ) Longitudinal scans of both lattice and magnetic order. Each peak is fit with a pseudo-Voigt function, in addition to an extra linear background for magnetic peaks ( g , h ). Vertical error bars represent 1 σ s.d. of counting statistics. The horizontal bars at the middle of each peak represent the FWHM of the instrument resolution. All intensities are normalized to that of the (0, 2, 0) Bragg peak. Full size image High-resolution X-ray diffraction We show in Fig. 1 representative scans of both the structural and magnetic order at high pressure and low temperature, P =16.1 GPa and T =5.2 K, exemplifying the high-resolution X-ray magnetic diffraction technique. GdSi has a collinear spin structure between the Néel temperature, T N =54.5 K, and the spin-flip transition temperature, T SF =53.0 K, and an orthorhombic lattice structure. Below T SF at ambient pressure, the spin structure is planar and is associated with a monoclinic lattice structure (space group P2 1 /c) that can be detected by a split of the d -spacing between (0, K , L ) and (0, K , − L ) [10] . There are then two magnetic domains with Q vectors along (0, ± q b , q c ) associated with the individual monoclinic lattice domains (see Fig. 1d and Fig. 2b , inset). At 16.1 GPa, the highest pressure that antiferromagnetism was directly observed, the monoclinic splitting of the (0, 1, 1) order remains clear ( Fig. 1f ), although the longitudinal line shapes are slightly broadened above the instrument resolution [21] . Here, both the spontaneously twinned single crystals and near-resolution-limited diffraction profiles testify to the quasi-hydrostatic pressure condition in the sample environment. At 16.1 GPa, the full widths at half maximum (FWHMs) of the peaks give a coherence length of 1,400 Å for both the lattice and the antiferromagnetic order. 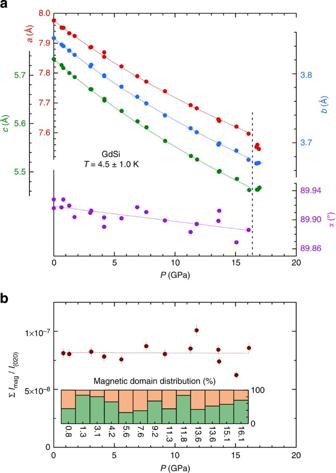Figure 2: Pressure dependence of both lattice structure and magnetic order parameter. (a) Lattice constants,a,b,c, and the monoclinic angleαas a function of pressure. BelowPc=16.4 GPa, lattice constantsa,b,care fit with the single-parameter Birch equation of state specified in the text.α(P) is fit linearly. AbovePc, there is a first-order structural transition to an orthorhombic phase. (b) The magnetic order parameterImag/I(020)is summed over diffraction intensities at (0, 2−qb, ±qc) and (0,qb, ±qc) for both magnetic domains. (Inset) Magnetic domain distribution at each pressure point where the order parameter was measured. Error bars represent 1σs.d. Figure 2: Pressure dependence of both lattice structure and magnetic order parameter. ( a ) Lattice constants, a , b , c , and the monoclinic angle α as a function of pressure. Below P c =16.4 GPa, lattice constants a , b , c are fit with the single-parameter Birch equation of state specified in the text. α ( P ) is fit linearly. Above P c , there is a first-order structural transition to an orthorhombic phase. ( b ) The magnetic order parameter I mag / I (020) is summed over diffraction intensities at (0, 2− q b , ± q c ) and (0, q b , ± q c ) for both magnetic domains. (Inset) Magnetic domain distribution at each pressure point where the order parameter was measured. Error bars represent 1 σ s.d. Full size image We plot in Fig. 2a the substantial change in the lattice constants with P . Each refined lattice constant, a , b and c , is fit with the single-parameter Birch equation of state: P =3/2 B l [( l 0 / l ) 7 −( l 0 / l ) 5 ], where l 0 is the individual lattice constant at ambient pressure. The three bulk moduli, B a =83.1±0.4 GPa, B b =88.0±0.3 GPa and B c =85.4±0.4 GPa, are close in value, indicating that the crystal structure evolves in a nearly isotropic fashion under pressure. Overall, the antiferromagnetism in GdSi persists over a 4.7% compression of the linear lattice constants and a 13% reduction in volume. At ambient pressure, the monoclinic angle α of the lattice tracks the evolution of the planar magnetic order via magnetostrictive coupling [10] . Up to 16.1 GPa, α changes only slightly and deviates slowly away from 90°. At a critical pressure, P c =16.4 GPa, the a -axis lattice constant shows a clear discontinuity of Δ a / a =5.9 × 10 −3 , while changes along the other two axes are minimal. Beyond P c , no splitting of the (0, K , L ) orders is observed for three different crystals as the lattice structure again becomes orthorhombic (the structure found for T>T SF at ambient pressure). The incommensurate antiferromagnetic order is no longer visible beyond P c , and the nature of the high-pressure phase, whether it is a paramagnet, a ferromagnet or a commensurate antiferromagnet, cannot be discerned from this data. Antiferromagnetic ground state under pressure The incommensurate antiferromagnetism in GdSi and its evolution with P can be probed directly by observing the magnetic order at points in reciprocal space such as (0, q b , ± q c ), (0, 2− q b , ± q c ) and (0, 2+ q b , ± q c ). The magnetic nature of these incommensurate diffraction peaks was demonstrated previously at ambient pressure via resonant X-ray diffraction, and no lattice (charge) coupling at this wave vector was detected [10] . As shown in Fig. 2b , and in telling contrast to the behaviour of the lattice, the magnetic order parameter remains unchanged over the entire range of pressures, 0≤P<P c =16.4 GPa. The magnetic order parameter was measured by summing over the diffraction intensities of both domains ( Fig. 2b , inset). In the diffraction geometry of a diamond anvil cell, it is difficult to measure a full azimuthal dependence under pressure [10] . However, given that the data were taken at a fixed azimuthal angle (see Methods), both the constant diffraction intensity and lattice monoclinic angle substantiate the interpretation that the spin structure is invariant under pressure. In addition to the strength of the magnetic order parameter, the stability of the incommensurate spin structure in GdSi under pressure is further illustrated through measurements of the wave vector Q . We show in Fig. 3 , Q ( P ) at fixed T and Q ( T ) at fixed P at the approaches to the quantum and thermal transitions, respectively. Along the temperature path, there is a significant change in Q ( T ) that accelerates near the phase boundary in a manner characteristic of many incommensurate SDW and CDW systems [8] , [22] . Under pressure, however, Q ( P ) of GdSi stays essentially constant (relative to the lattice) as it approaches the first-order, high-pressure phase boundary, with a slight, monotonic decrease in q b ( P ); the germane characteristics of the Fermi surface nesting are unaffected. We note that Q ( P ) would behave differently for systems approaching a continuous quantum phase transition. A non-monotonic Q ( P→P c ) has been measured in the incommensurate SDW in Cr arising from fluctuation effects at the approach to the quantum critical point [11] . Here, in GdSi, the magnetism does not weaken with applied pressure and quantum fluctuations have been cut off by the first-order structural transition. 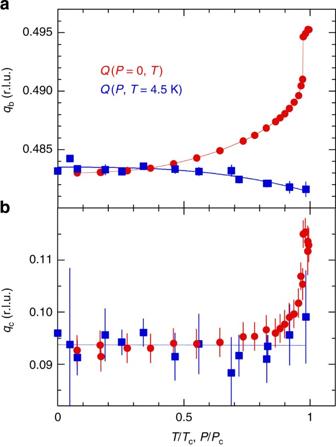Figure 3: Temperature and pressure dependence of the magnetic wave vector. (a,b) Evolution of the incommensurate wave vectorQ=(0,qb,qc) in reciprocal lattice unit (r.l.u.) towards the pressure- and temperature-induced phase boundaries. The Fermi surface nesting condition changes little withPat lowT. Horizontal axes are normalized byPcandTN, respectively. Error bars represent 1σs.d. Solid lines are guides to the eye. The discontinuity inQ(T) happens at the spin-flip transitionTSF. Figure 3: Temperature and pressure dependence of the magnetic wave vector. ( a , b ) Evolution of the incommensurate wave vector Q =(0, q b , q c ) in reciprocal lattice unit (r.l.u.) towards the pressure- and temperature-induced phase boundaries. The Fermi surface nesting condition changes little with P at low T . Horizontal axes are normalized by P c and T N , respectively. Error bars represent 1 σ s.d. Solid lines are guides to the eye. The discontinuity in Q ( T ) happens at the spin-flip transition T SF . Full size image Band structure calculations provide insight into the unusual hardiness of the incommensurate SDW in GdSi. At ambient pressure, the paramagnetic band structure of GdSi possesses four different itinerant bands at the Fermi surface. The band with the nested features takes up the majority of the density of states; the other three bands present as either small pockets or tubes. We plot in Fig. 4 projections and a three-dimensional perspective of the nested major band at four different pressures from 0 to 16.1 GPa (calculations for all the bands can be found in the Supplementary Fig. 1 ). This dominant band persists throughout the entire pressure range. The nesting condition is reinforced as the band gradually assumes a sheet-like shape at 16.1 GPa with a one-dimensional dispersion. A charge transfer effect slowly depletes its electronic density of states to the other minor bands. In addition, two extra bands start to emerge at the Fermi surface for pressures above 11 GPa, due to either charge transfer or bandwidth broadening ( Supplementary Fig. 1 ). However, the quasi-one-dimensional nesting vector—which would dominate the wave vector selection of the SDW—is essentially unchanged with pressure. 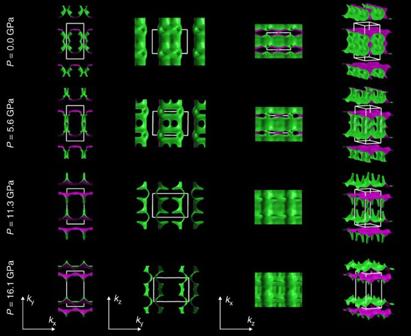Figure 4: Evolution of the nesting band under pressure. The calculated major itinerant band at the Fermi surface projected along each of three major reciprocal lattices, together with a three-dimensional perspective. The band structure calculations were carried out at four different pressures using the structural data ofFig. 2a. As pressure increases, a charge transfer process slowly depletes the band, but the nesting condition remains stable and grows progressively more one-dimensional. Figure 4: Evolution of the nesting band under pressure. The calculated major itinerant band at the Fermi surface projected along each of three major reciprocal lattices, together with a three-dimensional perspective. The band structure calculations were carried out at four different pressures using the structural data of Fig. 2a . As pressure increases, a charge transfer process slowly depletes the band, but the nesting condition remains stable and grows progressively more one-dimensional. Full size image Line-shape analysis of the resonant X-ray magnetic diffraction in GdSi at ambient pressure had illustrated the quasi-one-dimensional characteristics of the nested Fermi surface [10] . Between the two components of itinerant and local spins that collectively form the SDW, the localized Gd 4 f moments lie ~8 eV below the Fermi level [23] . In pure Gd, those 4 f spins would remain localized up to 106 GPa [15] . The stability of the antiferromagnetism in GdSi with P up to 16.4 GPa, as demonstrated by both its order parameter and its Q -vector, is then clearly connected to the stability of the nested itinerant band, which progressively becomes one-dimensional under pressure. Above that pressure, some mix of charge transfer and a first-order structural transition destroys the major nested band and cuts off the incommensurate SDW order in GdSi. The stability of antiferromagnetic order with large variations in the lattice spacing is unusual and raises fundamental physics and technological questions [20] . Very few examples exist in the literature for pressures above 10 GPa. High-pressure neutron powder diffraction on cubic Gd X ( X =Bi, Sb, As) compounds shows that antiferromagnetic order can survive to at least 17, 19.5 and 43 GPa, respectively [16] . These are commensurate orders of the (½, ½, ½) type that are locked into the lattice. For the incommensurate spin structure in GdSi, the stability in the hidden one-dimensional Fermi surface can be traced, at least in part, to particular features in the material’s structure. Although the magnetic order wave vector Q is incommensurate to both the b* and c* axes, it lies close to the b* direction. Sighting along the b axis ( Fig. 1a ), one sees Si atoms forming double chains inside a tubular Gd framework with a distorted hexagonal shape. This linear structural feature in real space is likely to be the source of the one-dimensional characteristics of the Fermi surface, as the band structure calculations reveal a strong character of Si carriers in the major nesting band. It is also instructive to compare the hidden one-dimensional SDW order in GdSi with correlated electron states in quasi-one-dimensional organic conductors such as TTF-TCNQ and (TMTTF) 2 X. The transition temperatures of all CDW, Spin–Peierls and antiferromagnetic/SDW states are generally found to vary slowly with pressure tuning [2] , [4] , [6] , except in narrow crossover regions between two different ground states [3] , [14] . Direct probes of the order parameter and wave vector evolution with P in these materials, presently very limited [24] , would be useful to explore the underlying characteristics of stability. More generally, organization principles that are robust against external disturbances—a generalized invar effect—provide opportunities for applications, ranging from giant magnetoresistance, multi-layer devices [25] to non-Abelian states in potential quantum computation applications [26] . In GdSi, the cooperative interaction between itinerant and local spin moments provides a robust magnetic ordering mechanism over a large strain range, which matches well with the typical range of elastic deformation for most functional materials [27] . Potentially, GdSi could be grown in thin film form, where the antiferromagnetism is expected to persist for significant lattice mismatches, and it could be a robust interfacial component in spin-valve and giant magnetoresistance devices [25] . The newly developed technical capability to examine directly incommensurate magnetism under tens of GPa pressure using X-ray magnetic diffraction provides a new means to continuously trace the interplay between spin, charge, itinerant and local degrees of freedom in functional materials. X-ray diffraction Non-resonant X-ray magnetic diffraction under pressure was performed at beamline 4-ID-D of the Advanced Photon Source [19] , [20] . A focused 20,000 keV X-ray beam was reduced to 100 × 100 μm 2 size by motorized slits to match typical sample sizes around 80 × 80 × 30 μm 3 under pressure. Miniature single-crystal GdSi samples were prepared in successive stages by cutting with electron discharge machining, polishing to final thickness and dicing with an infrared laser to final lateral dimensions. Additional specifications on sample growth can be found in ref. 10 . A NaI detector was used for measuring X-ray intensity, but no polarization analyser was used for magnetically diffracted X-rays. Using a six-circle Huber ψ-diffractometer in the vertical diffraction geometry, a high resolution in momentum space better than 1 × 10 −3 Å −1 FWHM is achieved for longitudinal scans [11] , [20] , [21] . All measurements were made at the base temperature of the cryostat, which varied between 3.5 and 5.5 K for various cooldowns. A total of seven samples were studied under pressure with three of them compressed across the phase transition. Complete data sets of both magnetic order parameter and wave vector were collected on four samples, although magnetic diffraction was observed on all six samples probed below P c . The magnetic order parameter was measured at a constant azimuthal angle ?=42°±2°, where ?=0 is for the azimuthal vector (0, 0, 1) inside the diffraction plane. This geometry provides sensitivity to spins aligned along both the a and c axes in the planar spin structure [10] . The Q vector is calculated through measured (0, 2+ q b , ± q c ), (0, 2− q b , ± q c ), (0, q b , ± q c ) and (0, 2, 0) orders, normalized to the lattice constants b and c at each P . High-pressure environment Pressure cells with conical Boehler–Almax type of diamond anvils (70° total 2θ angle) were used for single-crystal diffraction. We specifically designed a wide-angle ( 2θ =60°) partial perforation for all our diamond anvils ( Fig. 1a ). The partial perforation ends in a spherically curved shape (500 μm radius) to better distribute stress in the anvils under compression. A pair of these partially perforated anvils leaves 0.9 to 1.0 mm total diamond thickness in the X-ray path. By comparison with the typical total diamond thickness of 3.2–4.5 mm with normal anvils, this wide-angle partial perforation design significantly reduces the elastic X-ray scattering background, while still reaching at least 17 GPa for 800 μm culet-sized anvils. The pressure medium was a 4:1 methanol:ethanol solution, and the cells were equipped with a helium-membrane controlled in situ pressure tuning mechanism at low temperature [21] . At 16.1 GPa, the pressure inhomogeneity across our sample is estimated to be either 0.30 GPa FWHM using a comparison of the FWHM of lattice diffraction with that of the instrument resolution ( Fig. 1 ), accounting for the sample-specific bulk moduli [28] , or a full range of ±0.19 GPa from previous pressure chamber studies under similar conditions [21] . The pressure inhomogeneity is typically linearly proportional to the absolute pressure in our assembly [21] . Band structure calculations First-principle band structure calculations were performed in the WIEN2K implementation of the generalized gradient-approximation approach [29] using the full-potential linearized-augmented-plane-wave method [30] with local orbitals for a better variational flexibility in the radial basis functions [31] . For non-magnetic calculations, spin–orbit effects were taken into account using a second-order variational step using scalar-relativistic eigenfunctions as basis [32] . A modified tetragonal method [33] (with a k-mesh of 7 × 14 × 9) was used for the k-point integration in Brillouin zone. Plots of the Fermi surface were generated using XCRYSDEN [34] with code available from http://www.xcrysden.org/ . We also assumed all relative atomic positions are unchanged under pressure, and treated the lattice in the orthorhombic basis given the symmetry in the paramagnetic phase [10] . How to cite this article : Feng, Y. et al. Hidden one-dimensional spin modulation in a three-dimensional metal. Nat. Commun . 5:4218 doi: 10.1038/5218 (2014).